Scalable architecture for a room temperature solid-state quantum information processor The realization of a scalable quantum information processor has emerged over the past decade as one of the central challenges at the interface of fundamental science and engineering. Here we propose and analyse an architecture for a scalable, solid-state quantum information processor capable of operating at room temperature. Our approach is based on recent experimental advances involving nitrogen-vacancy colour centres in diamond. In particular, we demonstrate that the multiple challenges associated with operation at ambient temperature, individual addressing at the nanoscale, strong qubit coupling, robustness against disorder and low decoherence rates can be simultaneously achieved under realistic, experimentally relevant conditions. The architecture uses a novel approach to quantum information transfer and includes a hierarchy of control at successive length scales. Moreover, it alleviates the stringent constraints currently limiting the realization of scalable quantum processors and will provide fundamental insights into the physics of non-equilibrium many-body quantum systems. The majority of realistic approaches to quantum information processing impose stringent requirements on the qubit environment, ranging from ultra-high vacuum to ultra-low temperature [1] , [2] , [3] . Such requirements, designed to isolate the qubit from external noise, often represent major experimental hurdles and may eventually limit the potential technological impact of a quantum information processor. For these reasons, developing a realistic framework for a feasible solid-state quantum processor capable of operating at room temperature is of both fundamental and practical importance. Nitrogen-vacancy (NV) colour centres in diamond stand out among other promising qubit implementations [4] , [5] , [6] , [7] in that their electronic spins can be individually polarized, manipulated and optically detected under room-temperature conditions. Each NV centre constitutes an individual two-qubit quantum register as it also contains a localized nuclear spin. The nuclear spin, which has an extremely long coherence time, can serve as a memory qubit, storing quantum information, while the electronic spin can be used to initialize, read-out, and mediate coupling between nuclear spins of adjacent registers. Magnetic dipole interactions allow for coherent coupling between NV centres spatially separated by tens of nanometers. Although, in principle, a perfect array of NV centres would enable scalable quantum information processing, in practice, the finite creation efficiency of such centres, along with the requirements for parallelism, necessitate the coupling of registers separated by significantly larger distances. Recent advances involving the quantum manipulation of NV defects have allowed researchers to achieve sub-diffraction limited resolution, single-shot read-out, and dipole-coupling-mediated entanglement between neighbouring NV electronic spins [8] , [9] , [10] , [11] , [12] , [13] , [14] , [15] , [16] , [17] , [18] . Despite such substantial developments, it remains unclear whether these individual pieces, each of which invariably require a unique set of experimental conditions, can be seamlessly unified into a scalable room-temperature architecture [19] . Thus, the development of an architectural blueprint that combines the associated experimental facets, while demonstrating that such a combination can enable high-fidelity quantum operations, is of crucial importance. In what follows, we describe and analyse a feasible architecture for a room-temperature, diamond-based quantum information processor. Our approach makes use of an array of single NV centres, created through ion implantation and subsequent annealing [11] , [20] . To overcome the challenge of coupling remote NV registers, we develop a novel method that enables coherent long-range interactions between NV centres, mediated by an optically un-addressable 'dark' spin chain data bus (DSCB) [21] . For concreteness, within our architecture, we will consider the specific implementation of such a DSCB by utilizing implanted nitrogen impurities (P1 centres) with spin 1/2, as shown in Fig. 1a [8] , [22] . We analyse realistic imperfections and decoherence mechanisms, concluding that the implementation of this architecture is feasible with current experimental technology. Moreover, we demonstrate the possibility of high-fidelity remote coupling gates, whose error rates fall below the threshold for quantum error correction in a two-dimensional (2D) surface code [23] . 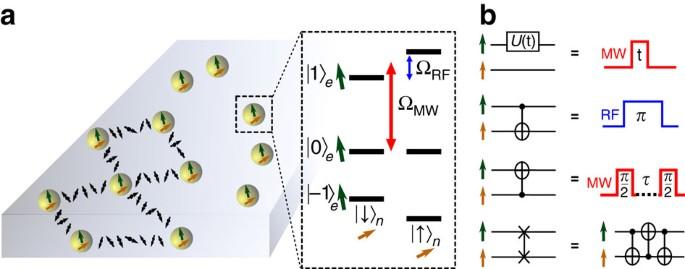Figure 1: Schematic representation of individual NV registers within bulk diamond. (a) Each NV register contains a nuclear spinI=1/2 (yellow), providing quantum memory, and an electronic spinS=1 (green). Dark spins (black) represent elements of an optically un-addressable spin chain, which coherently couples spatially separated NV registers. The NV level structure (in a high B field) is shown. A resonant MW (ΩMW) pulse coherently transfers the electronic spin of the register fromto; subsequent manipulation of the nuclear spin is accomplished through an RF pulse (ΩRF). The far detunedstate can be neglected to create an effective two-qubit register. However, the full three-level NV structure will be utilized in horizontal DSCB-mediated coherent coupling of NV registers. (b) A universal set of two-qubit gates can easily be achieved with only MW and RF controls26. Electronic spin manipulation can be accomplished with a MW field, wheretrepresents the duration of the MW pulse. By exploiting the hyperfine coupling between the electronic and nuclear spin, one can achieve controlled-NOT operations conditioned on either spin. In particular, a CeNOTngate can be accomplished by utilizing a RFπ-pulse, which flips the nuclear spin conditioned on the electronic spin being in |1〉e. Similarly, a CnNOTegate can be accomplished by utilizing the hyperfine interaction to generate a controlled-phase (CP) gate, whereτrepresents the duration of the wait time required to achieve such a hyperfine-driven CP gate. Performed between two single-qubit Hadamard gates (π/2-pulses) on the electronic spin, such a CP gate generates the desired CnNOTegate. Finally, combining the CeNOTnand CnNOTegates allows for the execution of a swap gate. Figure 1: Schematic representation of individual NV registers within bulk diamond. ( a ) Each NV register contains a nuclear spin I =1/2 (yellow), providing quantum memory, and an electronic spin S =1 (green). Dark spins (black) represent elements of an optically un-addressable spin chain, which coherently couples spatially separated NV registers. The NV level structure (in a high B field) is shown. A resonant MW (Ω MW ) pulse coherently transfers the electronic spin of the register from to ; subsequent manipulation of the nuclear spin is accomplished through an RF pulse (Ω RF ). The far detuned state can be neglected to create an effective two-qubit register. However, the full three-level NV structure will be utilized in horizontal DSCB-mediated coherent coupling of NV registers. ( b ) A universal set of two-qubit gates can easily be achieved with only MW and RF controls [26] . Electronic spin manipulation can be accomplished with a MW field, where t represents the duration of the MW pulse. By exploiting the hyperfine coupling between the electronic and nuclear spin, one can achieve controlled-NOT operations conditioned on either spin. In particular, a C e NOT n gate can be accomplished by utilizing a RF π -pulse, which flips the nuclear spin conditioned on the electronic spin being in |1〉 e . Similarly, a C n NOT e gate can be accomplished by utilizing the hyperfine interaction to generate a controlled-phase (CP) gate, where τ represents the duration of the wait time required to achieve such a hyperfine-driven CP gate. Performed between two single-qubit Hadamard gates ( π /2-pulses) on the electronic spin, such a CP gate generates the desired C n NOT e gate. Finally, combining the C e NOT n and C n NOT e gates allows for the execution of a swap gate. Full size image The NV qubit register Single NV registers contain a spin triplet electronic ground state ( S =1) and can be optically pumped and initialized to the spin state, which has no magnetic dipole coupling with other NV registers or impurities. After optical initialization, the electronic spin of each register remains in the state, unless coherently transferred to the state by a resonant microwave (MW) pulse, as shown in Fig. 1a [10] , [11] , [12] , [13] . The NV nuclear spin associated with nitrogen atoms ( I =1/2 for 15 N) possesses an extremely long coherence time ( 13 C nuclear spins could also in principle be utilized) and will serve as the memory qubit in our system [24] , [25] ; manipulation of the nuclear spin is accomplished with radio frequency (RF) pulses [26] . The Hamiltonian governing the electronic and nuclear spins of the NV register is with zero-field splitting Δ 0 =2.87GHz, electronic spin gyromagnetic ratio μ e =−2.8 MHz/Gauss, nuclear spin gyromagnetic ratio μ n =−0.43 kHz/Gauss, and hyperfine coupling A =3.0 MHz [10] . The application of a magnetic field along the NV-axis ( ) ensures full addressability of the two-qubit system, resulting in the energy levels shown in Fig. 1a . A universal set of two-qubit quantum operations can easily be achieved with only MW and RF controls, as shown in Fig. 1b and detailed in Methods [26] . Furthermore, it is possible to selectively read-out the state of the NV register; for example, to read-out the nuclear qubit of a register, we apply a C n NOT e gate to couple the electronic and nuclear spins, thereby allowing for read-out of the electronic spin based on fluorescence detection. Our approach to scalability will ultimately involve a hierarchical design principle that ensures a spatial separation between NV registers, which is of order the optical wavelength; while this will, in principle, enable individualized read-out, additional use of a red Laguerre-Gaussian donut beam can further enhance read-out fidelities [14] . Indeed, the read-out of individual registers may be complicated by the strong fluorescence background from neighbouring NV centres. To suppress this background fluorescence, a red donut beam can be used, with its minimum located at the particular NV centre being read-out [14] . Whereas the fluorescence signal from the NV register located at the minimum persists, the remaining illuminated registers will be dominated by the stimulated emission induced by the red donut beam. In addition to suppressing the background noise, the red donut beam can also suppress the nuclear decoherence of the remaining NV registers, by reducing the amount of time these registers spend in the electronic-excited state ( Supplementary Note 1 ) [27] . Moreover, this approach may be particularly applicable in the case where NV registers are separated by sub-optical-wavelength distances. After each round of fluorescence detection, the electronic spin is polarized to the state, while the I z component of the nuclear spin, a quantum non-demolition observable, remains unchanged [28] . Therefore, it is possible to repeat this read-out procedure multiple times to improve the read-out fidelity [15] , [16] . A strong magnetic field Tesla along the NV axis should be used to decouple the electronic and nuclear spins to achieve high-fidelity single-shot read-out of NV registers [16] . In addition to sub-wavelength read-out, optical donut beams also introduce the possibility of selectively manipulating individual NV registers with sub-wavelength resolution. In this case, we envision the use of a green Laguerre-Gaussian donut beam; whereas un-illuminated NV centres may respond to a resonant MW pulse, illuminated registers undergo a strong optical cycling transition that suppresses their response to MW pulses due to the quantum Zeno effect [29] , [30] . Approach to scalable architecture One of the key requirements for fault-tolerant quantum computation is the ability to perform parallel gate operations. In our approach, this is achieved by considering a hierarchy of controllability. The lowest level of the hierarchy consists of an individual optically addressable plaquette with horizontal and vertical spatial dimensions ∼ 100–500 nm, containing a single computational NV register, as shown in Fig. 2a . The plaquette dimensions are chosen such that register control and read-out can be achieved using conventional far-field or sub-wavelength optical techniques [10] , [14] , [24] , [30] , [31] . The second level, termed a super-plaquette ( ∼ 10 μm ×10 μm), consists of a lattice of plaquettes whose computational registers are coupled through DSCBs. At the highest level of the hierarchy, we consider an array of super-plaquettes, where individual super-plaquettes are controlled by confined MW fields [32] . In particular, micro-solenoids can confine fields to within super-plaquettes, allowing for parallel operations at the super-plaquette level. For example, as shown in Fig. 2 , independent MW pulses can allow for simultaneous operations on the electronic spins of all computational NV registers within all super-plaquettes. To control registers at the super-plaquette boundaries, we define a dual super-plaquette lattice ( Fig. 2a ). Localized MW fields, within such a dual lattice, can provide a smooth transition between the boundaries of neighbouring super-plaquettes. 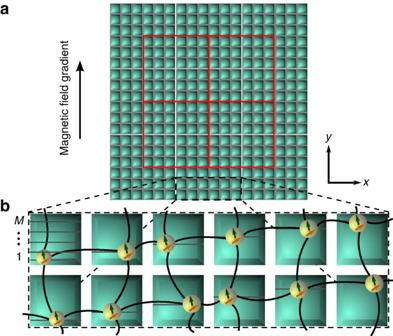Figure 2: The architecture for a room-temperature solid-state quantum computer. (a) A 2D hierarchical lattice allowing for length-scale-based control, which enables fully parallel operations. At the lowest level, individual plaquettes are outlined in grey and each contains a single computational NV register. At the second level of hierarchy, a super-plaquette, outlined in white, encompasses a lattice of plaquettes; each super-plaquette is separately manipulated by micro-solenoid confined MW fields. To allow for quantum information transfer across boundaries of super-plaquettes, there exists a dual super-plaquette lattice outlined in red. (b) The schematic NV register implantation within a super-plaquette. Two rows of individual plaquettes within a super-plaquette are shown. NV registers, consisting of an electronic (green) and nuclear (yellow) spin are shown within a staggered up-sloping array that is row-repetitive. Individual rows within a single plaquette are specified by an integernwithn=1 being the bottom row andn=Mbeing the top row. To achieve a staggered structure, we specify a unique implantation row within each plaquette wherein single impurities are implanted and subsequently annealed. For a given row of plaquettes, the implantation row corresponding to the left-most plaquette isn= 1, whereas the plaquette to the immediate right has implantation rown= 2; this pattern continues until the final plaquette in a given row, which by construction, has the highest implantation row number. The implantation process is repeated for each row of plaquettes within the super-plaquette and creates an array of NV registers, which each occupy a unique row in the super-plaquette. Because each NV register occupies a unique row within the super-plaquette, the magnetic field gradient in thedirection allows for individual spectroscopic addressing of single registers. Coherent coupling of spatially separated NV registers in adjacent plaquettes is mediated by a DSCB and is schematically represented by the curved lines connecting individual registers. The second implantation step corresponds to the creation of these horizontal and vertical dark spin chains. Figure 2: The architecture for a room-temperature solid-state quantum computer. ( a ) A 2D hierarchical lattice allowing for length-scale-based control, which enables fully parallel operations. At the lowest level, individual plaquettes are outlined in grey and each contains a single computational NV register. At the second level of hierarchy, a super-plaquette, outlined in white, encompasses a lattice of plaquettes; each super-plaquette is separately manipulated by micro-solenoid confined MW fields. To allow for quantum information transfer across boundaries of super-plaquettes, there exists a dual super-plaquette lattice outlined in red. ( b ) The schematic NV register implantation within a super-plaquette. Two rows of individual plaquettes within a super-plaquette are shown. NV registers, consisting of an electronic (green) and nuclear (yellow) spin are shown within a staggered up-sloping array that is row-repetitive. Individual rows within a single plaquette are specified by an integer n with n =1 being the bottom row and n = M being the top row. To achieve a staggered structure, we specify a unique implantation row within each plaquette wherein single impurities are implanted and subsequently annealed. For a given row of plaquettes, the implantation row corresponding to the left-most plaquette is n = 1, whereas the plaquette to the immediate right has implantation row n = 2; this pattern continues until the final plaquette in a given row, which by construction, has the highest implantation row number. The implantation process is repeated for each row of plaquettes within the super-plaquette and creates an array of NV registers, which each occupy a unique row in the super-plaquette. Because each NV register occupies a unique row within the super-plaquette, the magnetic field gradient in the direction allows for individual spectroscopic addressing of single registers. Coherent coupling of spatially separated NV registers in adjacent plaquettes is mediated by a DSCB and is schematically represented by the curved lines connecting individual registers. The second implantation step corresponds to the creation of these horizontal and vertical dark spin chains. Full size image Taking advantage of the separation of length scales inherent to optical control and MW confinement provides a mechanism to achieve parallelism; indeed, the hierarchical control of plaquettes, super-plaquettes and super-plaquette arrays allows for simultaneous single- and two-qubit gate operations, which are fundamental to fault-tolerant computation. One of the key differences between the currently proposed architecture and previous proposals [6] , [33] , is that the design here does not rely on optically resolved transitions, which are only accessible at cryogenic temperatures. The required 2D array of NV centres can be created via a two-step implantation process. We envision first implanting single nitrogen atoms along particular rows within each plaquette, as shown in Fig. 2b ; subsequent annealing occurs until the creation of an NV centre, after which, a second nitrogen implantation step generates the spin chain data bus. The selective manipulation of individual registers within our 2D array is enabled by the application of a spatially dependent external magnetic field ; this 1D magnetic field gradient is sufficiently strong ( α ∼ 10 5 T m −1 ) to allow for spectroscopic MW addressing of individual NV registers, each of which occupies a unique row in the super-plaquette, as shown in Fig. 2b [32] , [34] , [35] . Dark spin chain data bus To coherently couple two spatially separated NV centres, we consider two distinct approaches. First, we consider an approach, which is appropriate for spin-state transfer along the direction of the magnetic field gradient, in which individual addressing of spins is possible. This allows for an adiabatic sequential swap between neighbouring qubits and, consequently, between the ends of the chain. Alternatively, in the situation where individual addressing of spins is not possible (that is, in the direction transverse to the field gradient), we show that global control pulses achieve effective Hamiltonian evolution, which enables quantum state transfer through the spin chain. In both cases, we show that perfect state transfer and remote coupling gates are possible even when the intermediate spin chain is completely unpolarized (infinite spin temperature). We begin by analysing the adiabatic sequential swap in a spin-1/2 chain. This approach is suitable to couple registers in plaquettes that are vertically adjacent, relying on the individual addressability of qubits and utilizing the magnetic dipole coupling between spin-chain elements. As shown in the Supplementary Methods , under the secular approximation, the magnetic dipole coupling between a pair of neighbouring spins can be reduced to Ising form where κ is the relevant component of the dipole tensor, ω 0 captures the electronic Zeeman energy, and δ i characterizes both the hyperfine term (nuclear spin dependent) and the magnetic field gradient. From the Ising Hamiltonian, an XX interaction between qubits can be distilled by driving with , leading to (under the rotating wave approximation, in the rotating frame, with , and in a rotated basis with ( x , y , z )→( z , − y , x )) The spin-flip process in H int is highly suppressed in the limit of , whereas the same process is dominant in the case of . Hence, by slowly ramping the Rabi frequencies Ω 1 and Ω 2 through one another, adiabatic swap of the quantum states of the two impurities can be achieved through rapid adiabatic passage, as shown in Fig. 3a . Generalizing to arbitrary length spin chains yields , whereby the sequential adiabatic swap of quantum states along the spin chain can be achieved by successively tuning individual Rabi frequencies across one another. During the adiabatic swap of a single pair of spins, higher order interactions, such as those resulting from next-to-nearest neighbours, will be suppressed because of the differences in Rabi frequencies. By including the magnetic dipole coupling between the electronic spin of the NV register and the spin chain quantum channel, we arrive at an effective mixed spin chain with the DSCB connecting the two electronic spins of the vertically separated NV registers. 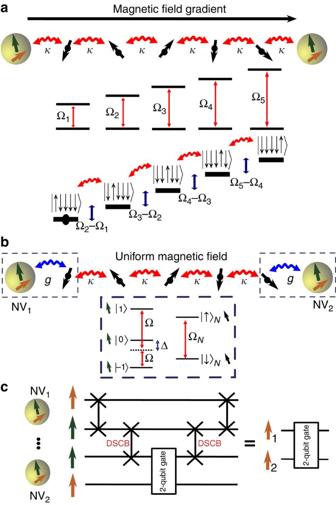Figure 3: DSCB-mediated coherent coupling of spatially separated NV registers. (a) Adiabatic sequential swap along the vertical direction, parallel to the magnetic field gradient. Individual addressing of impurities, enabled by the field gradient, allows for a slow ramping of the Rabi frequencies Ωiand Ωjthrough one another; this achieves adiabatic swap of the quantum states of the two impurities through rapid adiabatic passage. Thus, sequential adiabatic swap of quantum states along the spin chain can be achieved by successively tuning individual Rabi frequencies across one another. (b) FFST in the horizontal direction, transverse to the magnetic field gradient. The coupling strength between the end qubits and the spin chain isg, whereas the interchain coupling strength isκ. Schematic representation of the level structure of the NV electronic spin and a dark impurity spin. Controlling the NV-impurity couplinggis an essential component of FFST and occurs by driving the NV in two-photon resonance, with Rabi frequency Ω and detuning Δ. (c) Schematic circuit diagram outlining the protocol to achieve coherent coupling between the nuclear memory qubits of spatially separated NV registers. First, the nuclear and electronic qubits of a single register are swapped. Next, the electronic qubits of the two NV centres to be coupled are swapped through the DSCB. Finally, a two-qubit gate between the electronic and nuclear spin of the second register is performed, before the memory qubit is returned to the nuclear spin of the original NV centre. Figure 3: DSCB-mediated coherent coupling of spatially separated NV registers. ( a ) Adiabatic sequential swap along the vertical direction, parallel to the magnetic field gradient. Individual addressing of impurities, enabled by the field gradient, allows for a slow ramping of the Rabi frequencies Ω i and Ω j through one another; this achieves adiabatic swap of the quantum states of the two impurities through rapid adiabatic passage. Thus, sequential adiabatic swap of quantum states along the spin chain can be achieved by successively tuning individual Rabi frequencies across one another. ( b ) FFST in the horizontal direction, transverse to the magnetic field gradient. The coupling strength between the end qubits and the spin chain is g , whereas the interchain coupling strength is κ . Schematic representation of the level structure of the NV electronic spin and a dark impurity spin. Controlling the NV-impurity coupling g is an essential component of FFST and occurs by driving the NV in two-photon resonance, with Rabi frequency Ω and detuning Δ. ( c ) Schematic circuit diagram outlining the protocol to achieve coherent coupling between the nuclear memory qubits of spatially separated NV registers. First, the nuclear and electronic qubits of a single register are swapped. Next, the electronic qubits of the two NV centres to be coupled are swapped through the DSCB. Finally, a two-qubit gate between the electronic and nuclear spin of the second register is performed, before the memory qubit is returned to the nuclear spin of the original NV centre. Full size image Crucially, such an adiabatic sequential swap is robust against variations in the coupling strength κ , which can be induced by the imprecise implantation of impurities that form the spin-1/2 chain; in particular, even for the case of varying κ i , i +1 , perfect adiabatic swap occurs so long as the rate at which Ω i and Ω i +1 are ramped through one another is sufficiently small. Within the proposed architecture, the impurities forming the horizontal spin chain will not induce operational errors during the vertical adiabatic sequential swap as the design principle allows for selective spin echoing (Fig. 5). Next, we consider a second method, termed free-fermion state transfer (FFST) developed in ref. 36 , to coherently couple NV registers in the horizontal direction. In contrast to the adiabatic sequential swap, the method utilizes only global control over dark impurities and effective Hamiltonian evolution. The relaxation of the requirement of individual control over elements of the dark spin chain renders this second method, applicable for coherent coupling between NV registers in horizontally adjacent plaquettes, transverse to the direction of the field gradient. In particular, the protocol achieves coherent coupling through an unpolarized, infinite-temperature spin chain, employing purely Hamiltonian evolution under as shown in Fig. 3b . This Hamiltonian, obtained in a similar fashion equation (3), results in coherent interactions between NV centres, which is best understood through an analogy with eigenmode tunneling in a many-body system. Specifically, the spin chain described by H FFST can be viewed as a system of non-interacting fermions. As described in ref. 36 , by tuning the NV centres into resonance with a single fermionic eigenmode, an effective three-state system can be realized. Mediated by this fermionic eigenmode, the electronic states of two remote NV centres can be coherently swapped. Coupled with arbitrary two-qubit gates between the nuclear and electronic spin ( Fig. 1b ; Methods), an electronic swap gate enables universal computation between spatially remote nuclear spin memories, as shown in Fig. 3c . Crucially, such a swap gate is insensitive to the polarization of the intermediate dark spins and high-fidelity quantum state transfer can be achieved, provided that the fermionic mode is delocalized and that the coupling, g , of the NV qubit to the spin chain is controllable. As detailed in the Methods, by utilizing the three-level NV ground-state structure ( Fig. 3b ), it is possible to fully control the NV-chain coupling. This tunability also ensures that FFST is fundamentally robust to experimentally relevant coupling-strength disorder, which could be induced by implantation imprecision. Indeed, by separately tuning the NV-chain coupling on either side of the DSCB, it is possible to compensate for both disorder-induced asymmetry in the fermionic eigenmode as well as altered eigenenergies ( Supplementary Methods ) [36] , [37] , [38] . Implementation, operational errors and gate fidelities The specific implementation of the DSCB can be achieved with implanted nitrogen impurity ions. Dipole coupling between neighbouring nitrogen electronic spins forms the DSCB, whereas dipole coupling between the NV and nitrogen electronic spins forms the qubit–DSCB interaction; non-secular terms of this magnetic dipole coupling are highly suppressed owing to the spatially dependent external magnetic field B z ( y ), resulting in the effective interaction found in equation (2). In addition, the nitrogen impurities possess a strong hyperfine coupling, the principal axis of which can take on four possible orientations due to tetrahedral symmetry [39] , [40] , [41] . Dynamic Jahn–Teller (JT) reorientation of the nitrogen impurity's hyperfine principal axis results in two particular considerations, namely the addressing of additional JT frequencies yielding a denser super-plaquette frequency spectrum and the JT-governed spin-lattice relaxation time ( Supplementary Methods ). As is characterized by an Arrhenius rate equation [40] at ambient temperatures, a combination of a static electric field and slight cooling by ∼ 50 K allows for a substantial extension of the relaxation time to ∼ 1 s; hence, in the following consideration of operational errors, we will assume that we are limited by , the spin-lattice relaxation time of the NV centre. We now consider various imperfections, which may introduce operational errors. In particular, we consider the errors associated with the sequential swap-mediated coupling between vertically adjacent registers and the FFST between horizontally adjacent registers. We begin by discussing the analytic error estimate associated with each method, after which, we summarize the results of full numerical simulations ( Supplementary Methods ). First, we consider the accumulated infidelity associated with the adiabatic sequential swap, The first term, , represents off-resonant cross-talk induced by MW manipulations with Rabi frequency Ω i . Here Δ g characterizes the gradient-induced splitting achieved within the super-plaquette frequency spectrum ( Supplementary Methods ). The second term, p adia , corresponds to the non-adiabatic correction resulting from an optimized adiabatic ramp profile [42] , [43] , [44] . The third term, , is directly obtained from equation (3) and corresponds to additional off-resonant errors. The fourth error term, corresponds to the depolarization error induced by the finite NV T 1 time, while the final error term, corresponds to the infidelity induced by dephasing. As each error term is considered within the context of a single adiabatic swap, the total error contains an additional factor of N , representing the chain length, which is plaquette size dependent. We can similarly consider the accumulated infidelity associated with FFST, In direct analogy to , the first term in corresponds to the excitation of an NV register by off-resonant MW fields. The second term, p f , corresponds to the undesired coupling with off-resonant fermionic modes. Since the coupling strength is characterized by [36] , while the splitting of the eigenenergy spectrum ∼ κ / N , such an off-resonant error induces an infidelity . The third error term, p g , results from the protocol designed to control, g , the NV-chain coupling (see Methods for details). Directly analogous to , the fourth and fifth terms correspond to errors induced by the operational time, t FFST , which causes both depolarization and dephasing. Finally, we perform numerical simulations, taking into account the nitrogen JT frequencies, to characterize the infidelity of both the adiabatic sequential swap and FFST within the NV architecture, as shown in Fig. 4 . The results of these calculations are in excellent agreement with the above theoretical predictions. In particular, these simulations reveal that, for sufficiently long , operational infidelities in both DSCB methods can be kept below 10 −2 . 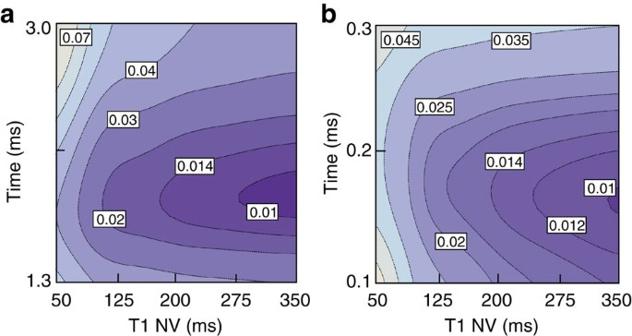Figure 4: Numerical simulation of the DSCB fidelity. (a) The operational infidelity associated with the adiabatic sequential swap forN=18. The simulations account for the JT orientation of nitrogen impurities and utilize the optimized adiabatic ramp profile42. Simulations utilize an optimized coupling strength of 8.71 kHz (18.1 nm spacing). Full numerical integration of the time-dependent Schrödinger equation produces infidelity contour plots as a function of total swap time and. (b) Numerical simulations of the operational infidelity associated with FFST forN=7. Non-nearest neighbour interactions are assumed to be refocused through dynamic decoupling as described in the Methods. Simulations, which utilize an optimized coupling strength of 12.6kHz (16 nm spacing), are based on a full diagonalization and also account for the JT orientation of nitrogen impurities. Infidelity contour plots are again shown as a function of total swap time and. Figure 4: Numerical simulation of the DSCB fidelity. ( a ) The operational infidelity associated with the adiabatic sequential swap for N =18. The simulations account for the JT orientation of nitrogen impurities and utilize the optimized adiabatic ramp profile [42] . Simulations utilize an optimized coupling strength of 8.71 kHz (18.1 nm spacing). Full numerical integration of the time-dependent Schrödinger equation produces infidelity contour plots as a function of total swap time and . ( b ) Numerical simulations of the operational infidelity associated with FFST for N =7. Non-nearest neighbour interactions are assumed to be refocused through dynamic decoupling as described in the Methods. Simulations, which utilize an optimized coupling strength of 12.6kHz (16 nm spacing), are based on a full diagonalization and also account for the JT orientation of nitrogen impurities. Infidelity contour plots are again shown as a function of total swap time and . Full size image These simulations clearly show that the T 1 time of the NV electronic spin is of critical importance in obtaining high-fidelity quantum operations. While at room temperature, T 1 appears to vary depending on the particular sample and on the specific properties of the local NV environment, such as strain, values on the order of 10 ms are generally obtained [24] , [39] . However, the spin-lattice relaxation mechanism governing T 1 is most likely related to an Orbach process [45] , [46] , which is strongly temperature dependent. In such a case, modest cooling of the sample by ∼ 50 K, is likely to extend T1 by more than an order of magnitude, thereby making high-fidelity gates possible. Given that such numerical estimations suggest the possibility of achieving high-fidelity two-qubit operations between remote NV registers, the proposed architecture seems well suited to the implementation of topological quantum error correction. In particular, we imagine implementing a 2D surface code, which requires only nearest-neighbour two-qubit gates and single-qubit preparation and measurement [23] , [47] , [48] . Recent progress in optimizing this surface code has yielded an error threshold of ɛ ∼ 1.4% (ref. 49 ), which is above the estimated infidelity corresponding to both the adiabatic sequential swap and FFST; thus, in principle, implementation of such a 2D surface code can allow for successful topological quantum error correction, and hence, fault tolerant quantum computation [50] . The above considerations indicate the feasibility of experimentally realizing a solid-state quantum computer capable of operating under ambient conditions at or near room temperature. We emphasize that a majority of the elements required for the realization of individual qubits in our architecture have already been demonstrated. In our approach, these techniques are supplemented by both a new mechanism for remote register coupling between NV centres as well as a hierarchical design principle, which facilitates scalability. The remote coupling mechanisms discussed can naturally be implemented via nitrogen ion implantation in ultra-pure diamond crystals and are robust to realistic imperfections and disorder [36] . Moreover, single errors during quantum state transfer are localized to individual transport channels and do not have a propagating effect on the remaining computation. While we hope that the proposed architecture evinces the feasibility of room temperature quantum information processing, the implementation and integration of the various proposed elements still require significant advances in areas ranging from engineering to materials science. Crucially, recent results have demonstrated substantial progress towards overcoming challenges such as the optimization of planar microcoil arrays [51] , [52] and efficient beam steering in micromirror systems [53] . Furthermore, by eliminating requirements for cryogenic temperatures, our blueprint aims to make the realization of a scalable quantum computer significantly more practical. The present work opens a number of new directions that can subsequently be explored. In particular, although we have considered the direct errors associated with DSCB-mediated coupling, it is instructive to note that the fidelity of such quantum gates can often be significantly improved, using techniques from optimal control theory [54] , [55] . For example, such methods of optimal control, while negating the detrimental effects of decoherence, can also simultaneously allow for the implementation of high-fidelity gates, despite both frequency and coupling disorder as induced by ion implantation errors. Indeed, the ability to precisely guide the quantum evolution via optimal control, even when the system complexity is exacerbated by environmental coupling, provides an alternative solution to improve single- and two-qubit gate fidelities [56] . In addition, it is well known that the local strain field surrounding each NV centre can significantly alter the register's properties; hence, through a detailed understanding of electric field induced strain, it may be possible to improve the coherence properties of the qubit. Moreover, the long coherence times of individual P1 centres, each of which harbours an associated nuclear spin, suggest the possibility of utilizing these dark spins as computational resources in and of themselves [57] . Beyond these specific applications, a number of scientific avenues can be explored, including, for example, understanding and controlling the non-equilibrium dynamics of disordered spin systems. Controlling qubit-chain coupling in the NV architecture To achieve an effective Hamiltonian of the form given by equation (4), it is essential to control the coupling strength between the NV register and the neighbouring impurity. Here we utilize the three levels of the NV electronic spin [58] to effectively control g , as shown in Fig. 3b , whereby the Hamiltonian (under MW driving) can be written as where Ω represents the Rabi frequency on the NV register, Δ represents the associated detuning, and Ω N represents the Rabi frequency on the nitrogen impurity. In this case, as the NV two-photon detuning is zero, it is convenient to define bright and dark states, and ; further, in the resulting two-level picture, the associated dressed states are and , in the limit . Hence, rewriting the Hamiltonian in this limit yields where correspond to the two -eigenstates of the nitrogen impurity. The coupling term can be further re-expressed as Thus, by working within the NV subspace {| D 〉,|−〉}, it is possible to completely control the coupling between the NV register and Nitrogen impurity, , by tuning the Rabi frequency and detuning. It is possible to work in the required two-state subspace by ensuring that and hence, that the |+〉 state remains unpopulated, with corresponding off-resonant error κ 2 /Δ 2 . Furthermore, we evince a possible scheme to coherently map the quantum information that is stored in the nuclear memory into the desired electronic subspace. For example, consider mapping |0〉 ( α |↑〉+ β |↓〉) to ( α |−〉+ β | D 〉) |↑〉, where the first (tensor) factor corresponds to the electronic state and the second corresponds to the nuclear state of a single NV. The proposed mapping can be achieved in a two-step process. First, by simultaneously performing a π −pulse on the transitions |0〉 |↓〉→|−1〉 |↓〉 and |0〉 |↓〉→|1〉 |↓〉 with oppositely signed Rabi frequencies, one can map |0〉 |↓〉 to | D 〉 |↓〉. Next, one utilizes an RF pulse to flip the nuclear spin, which yields | D 〉 |↓〉→| D 〉 |↑〉. Finally, turning Ω on in an adiabatic fashion ensures that the state preparation populates only | D 〉 and |−〉, thereby mapping the quantum information into the desired electronic subspace. Arbitrary two-qubit gates within the NV register Whereas the DSCB enables long-range quantum logic between spatially separated NV electronic spins, universal two-qubit gates between the nuclear spin quantum memories require additional local logic between nuclear and electronic spins, as outlined in Fig. 1b . Here we specify, in detail, the implementation of such local logic gates. A strong MW pulse (with ) can perform an arbitrary electronic spin rotation independent of the nuclear spin state. This can be mapped to a nuclear spin rotation by implementing a swap gate between the nuclear and electronic spins. Such a swap gate can be decomposed into three controlled-NOT gates: C e NOT n C n NOT e C e NOT n . A C e NOT n gate can be accomplished by utilizing an RF π -pulse (with ), which flips the nuclear spin conditioned on the electronic spin being in |1〉 e . Finally, a hyperfine-driven controlled-phase gate enables the remaining C n NOT e gate (up to single Hadamards on the electronic spin). This demonstrates that a universal set of local two-qubit gates between NV electronic and nuclear spins can easily be achieved with only MW and RF controls [26] . Such arbitrary local logic is crucial to enable the preparation of nuclear spin quantum information and forms an important portion of DSCB-mediated remote coupling ( Fig. 3c ). Specific implementation of architecture In this section, we offer a specific implementation of the architectural design principle and discuss the various ingredients required to achieve DSCB-mediated coherent coupling between spatially separated NV registers. In particular, we consider the refocusing of non-nearest neighbour interactions along the horizontal spin chain. The effective Hamiltonian evinced in equation (4) has nearest neighbour form; although next-nearest-neighbour interactions will represent a correction, we show that such interactions can be refocused within the current architectural design, and further, that, in principle, interactions beyond next-nearest-neighbour can also be refocused. In particular, the horizontal spin chain ( N total spins) is arranged in a staggered saw-tooth fashion, as shown in Fig. 5 . 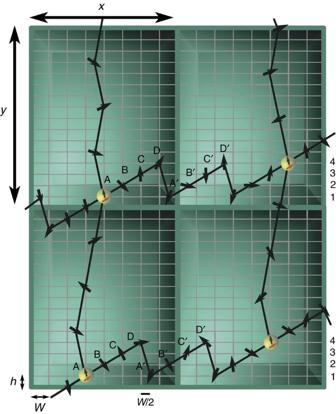Figure 5: Schematic Architectural Design. Specific impurity implantation within the architecture, which is designed to achieve parallel gate operations. Plaquettes, outlined in green, are chosen withy∼600 nm andx∼550 nm; the individual plaquette-lattice spacing is chosen withh∼6 nm andw∼20 nm. The magnetic field is oriented along the NV axis, which is normal to the shown computational plane (Supplementary Fig. S1) and the gradient is represented by the change in this field strength along thedirection. The distance between all nearest-neighbour pairs in the horizontal direction is∼21 nm () and thespacing between spinDand spinA′is given byw/2. We note that the figure is not drawn to scale and that all impurity spins sit on the horizontal lattice, whereas some impurity spins sit at midpoints of the vertical lattice. The particular lattice spacing is chosen to ensure that the spatial separation between individual nitrogen impurities forming the spin chain, as well as between NV registers and nitrogens does not exceed∼20 nm. The chosen plaquette-lattice spacing implies that neighbouring plaquettes are coupled by∼25 nitrogen impurities (black spins) in thedirection and by∼30 nitrogen impurities in thedirection. The zig–zag pattern of impurity implantation in thedirection (w/2 horizontal distance) ensures that all spin chain links are of identical length, thereby allowing for parallel sequential swap operations along. Additionally, such a pattern overcomes the limitation of imperfect NV conversion efficiency (Supplementary Note 2) by allowing each vertical spin chain to span a sufficiently large horizontal spacing. As the impurities forming the horizontal spin chain occupy unique rows relative to the vertical spin chain, during the adiabatic sequential swap, selective spin echoing of the horizontal chain impurities ensures that dipole coupling from such impurities will not induce operational errors. While the architecture is designed to showcase the ability to utilize the adiabatic sequential swap and FFST in differing directions, it is important to note that within the specific blueprint above, either implementation of the DSCB can be used in both directions. Within such an architecture, nearest neighbour coupling terms correspond to all pairs of adjacent spins, each separated by ∼ 20 nm, with corresponding interaction Hamiltonian Figure 5: Schematic Architectural Design. Specific impurity implantation within the architecture, which is designed to achieve parallel gate operations. Plaquettes, outlined in green, are chosen with y ∼ 600 nm and x ∼ 550 nm; the individual plaquette-lattice spacing is chosen with h ∼ 6 nm and w ∼ 20 nm. The magnetic field is oriented along the NV axis, which is normal to the shown computational plane ( Supplementary Fig. S1 ) and the gradient is represented by the change in this field strength along the direction. The distance between all nearest-neighbour pairs in the horizontal direction is ∼ 21 nm ( ) and the spacing between spin D and spin A ′ is given by w /2. We note that the figure is not drawn to scale and that all impurity spins sit on the horizontal lattice, whereas some impurity spins sit at midpoints of the vertical lattice. The particular lattice spacing is chosen to ensure that the spatial separation between individual nitrogen impurities forming the spin chain, as well as between NV registers and nitrogens does not exceed ∼ 20 nm. The chosen plaquette-lattice spacing implies that neighbouring plaquettes are coupled by ∼ 25 nitrogen impurities (black spins) in the direction and by ∼ 30 nitrogen impurities in the direction. The zig–zag pattern of impurity implantation in the direction ( w /2 horizontal distance) ensures that all spin chain links are of identical length, thereby allowing for parallel sequential swap operations along . Additionally, such a pattern overcomes the limitation of imperfect NV conversion efficiency ( Supplementary Note 2 ) by allowing each vertical spin chain to span a sufficiently large horizontal spacing. As the impurities forming the horizontal spin chain occupy unique rows relative to the vertical spin chain, during the adiabatic sequential swap, selective spin echoing of the horizontal chain impurities ensures that dipole coupling from such impurities will not induce operational errors. While the architecture is designed to showcase the ability to utilize the adiabatic sequential swap and FFST in differing directions, it is important to note that within the specific blueprint above, either implementation of the DSCB can be used in both directions. Full size image where the sum runs over all nearest neighbour pairs in a given dark spin chain. Thus, next-to-nearest neighbour terms for each spin correspond to the subsequent strongest interaction where the prime denotes the next link in the saw-tooth chain as shown in Fig. 5 . In addition to the impurity spins, FFST incorporates the electronic spin of the NV register into a mixed spin chain. It is important to note that the spin-flip Hamiltonians H N and H NN are derived from the secular approximated Ising coupling by the application of driving fields as per equation (3). As each row (1,2,3,4) is separately addressable by virtue of the magnetic field gradient (applying four frequencies per row to ensure that all JT and nuclear spin states are addressed), it is possible to apply a spin-echo procedure to refocus the next-nearest-neighbour terms. In particular, by flipping the spins in rows 1 and 2 ( Fig. 5 ) after time T d /2, where T d is a small fraction of the desired evolution duration, the next-nearest-neighbour interactions are refocused since each term contains spins from only row 1 or 2. However, half of the nearest neighbour interactions are also refocused, leaving effective evolution under the Hamiltonian Analogously, by flipping the spins in rows 2 and 3, effective evolution under the Hamiltonian is achieved, again with H NN refocused. Combining the evolution according to H eff 1 and H eff 2 yields the desired nearest-neighbour Hamiltonian with next-to-nearest neighbour interactions refocused. However, as H eff 1 and H eff 2 do not commute, it will be necessary to employ piecewise evolution according to the Trotter–Suzuki formalism [59] . Further refocusing of higher order non-nearest neighbour interactions can also be achieved by extending the number of rows corresponding to the saw-tooth design; such an extension allows for the isolation of each specific pair of nearest neighbour interactions, thereby achieving the desired nearest-neighbour evolution through a Trotter sequence. How to cite this article: Yao, N. Y. et al . Scalable architecture for a room temperature solid-state quantum information processor. Nat. Commun . 3:800 doi: 10.1038/ncomms1788 (2012).